Room-temperature spin-spiral multiferroicity in high-pressure cupric oxide Multiferroic materials, in which ferroelectric and magnetic ordering coexist, are of fundamental interest for the development of multi-state memory devices that allow for electrical writing and non-destructive magnetic readout operation. The great challenge is to create multiferroic materials that operate at room temperature and have a large ferroelectric polarization P . Cupric oxide, CuO, is promising because it exhibits a significant polarization, that is, P ~0.1 μC cm −2 , for a spin-spiral multiferroic. Unfortunately, CuO is only ferroelectric in a temperature range of 20 K, from 210 to 230 K. Here, by using a combination of density functional theory and Monte Carlo calculations, we establish that pressure-driven phase competition induces a giant stabilization of the multiferroic phase of CuO, which at 20–40 GPa becomes stable in a domain larger than 300 K, from 0 to T> 300 K. Thus, under high pressure, CuO is predicted to be a room-temperature multiferroic with large polarization. Since the first observation of multiferroicity [1] , [2] in cupric oxide (CuO) by Kimura et al . [3] , it has been established that CuO is a type-II multiferroic, so that ferroelectricity occurs as a result of magnetic ordering [3] , [4] and, therefore, the multiferroic ordering temperature equals the magnetic ordering temperature T N =230 K. Moreover, CuO is a quasi-one-dimensional (1D) magnetic system with a large magnetic coupling J z ~80 meV (refs 5 , 6 , 7 ), which explains the high ordering temperature T N . In addition, upon cooling, a polar incommensurate antiferromagnetic (AF) spin-spiral ordering, referred to as AF 2 , appears below T N =230 K and a non-polar commensurate AF spin structure, AF 1 , below the lock-in temperature T L =213 K. Finally, the Dzyaloshinskii–Moriya (DM) ‘cycloidal’ interactions have been shown to have a major role in the emergence of the electric polarization in CuO [8] , [9] , [10] . Different aspects of the interplay between the magnetic, orbital and electronic degrees of freedom in CuO have been studied intensely [8] , [9] , [10] , [11] , [12] , [13] , [14] . Recently, we have shown that by applying a pressure of 8.8 GPa to CuO [14] , the magnetic exchange interactions can increase by 46%. This holds the promise that under pressure T N will increase, perhaps even to room temperature (RT). Indeed, the monoclinic phase of CuO is known to be stable up to at least 70 GPa [15] , even if detailed structural refinements are only available at pressures lower than 10 GPa [16] . Establishing the stability of the multiferroic phase under pressure, this topic not only requires a calculation of the magnetic exchange interactions by density functional theory (DFT) but also a determination of T L , T N and the temperature dependence of the polarization P by complementary methodologies. Here we establish that pressure-driven phase competition renders CuO multiferroic at RT with a large P . For this, we employ both a semi-empirical ansatz as well as unbiased classical Monte Carlo (MC) simulations. More specifically, using a combination of DFT and MC calculations, we demonstrate that upon applying pressure the effective magnetic dimensionality initially decreases, passes through a minimum and subsequently increases, the magneto-crystalline anisotropy (MAE) is reduced and the stability range of the multiferroic state strongly increases by lowering T L and increasing T N . Pressure effect on the magnetic exchange parameters CuO consists of corner- and edge-sharing square-planar CuO 4 units, which form (–Cu–O–) ∞ zigzag chains running along the [10–1] and [101] directions of the unit cell [17] . The low-T magnetic structure, AF 1 , consists of Cu moments arranged antiferromagnetically along [10–1] and ferromagnetically along [101], with the [010] direction as the easy axis [18] . The exchange interactions are captured by the Heisenberg Hamiltonian H H =∑ ij J ij S i · S j , which, to properly describe the magnetic properties of CuO, requires at least five magnetic exchange coupling parameters, that is, four superexchange interactions ( J a , J b , J x and J z ) and one super-superexchange interaction ( J 2a ) [7] , [14] , [19] , [20] (see Fig. 1a ). The pressure dependence of the unit cell volume and of the J -values is shown in Fig. 1b, c , respectively. 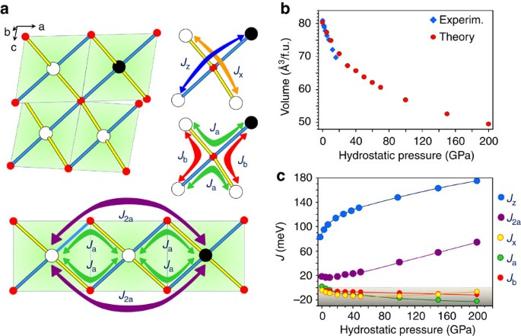Figure 1: High-pressure evolution of the structural and magnetic properties of CuO. (a) Schematic view of the tetrahedral environment of oxygen atoms in CuO and definition of the largest (Jz) and smaller magnetic superexchange couplings (Jx,JaandJb). The super-superexchange magnetic coupling,J2a, corresponds to the second-neighbour interaction of the edge-sharing chains, defined by the first-neighbour interaction,Ja. Oxygen atoms are represented by small red dots, and the Cu2+sites are depicted as filled and open dots, representing up-spin and down-spin, respectively. (b) Pressure dependence of the volume of CuO. The experimental values, deduced from a Birch–Murnaghan equation of state fitted to data of nanocrystalline CuO up to a pressure of 17 GPa (ref.21), are compared with those calculated by DFT. (c) Pressure dependence of the magnetic exchange couplings of CuO. Positive and negative values represent antiferromagnetic and ferromagnetic interactions, respectively. TheJ’s in the grey area are ferromagnetic. The uncertainty in the DFTJijvalues is between 1.2 and 2.5 meV (that is, smaller than the symbols). Figure 1: High-pressure evolution of the structural and magnetic properties of CuO. ( a ) Schematic view of the tetrahedral environment of oxygen atoms in CuO and definition of the largest ( J z ) and smaller magnetic superexchange couplings ( J x , J a and J b ). The super-superexchange magnetic coupling, J 2a , corresponds to the second-neighbour interaction of the edge-sharing chains, defined by the first-neighbour interaction, J a . Oxygen atoms are represented by small red dots, and the Cu 2+ sites are depicted as filled and open dots, representing up-spin and down-spin, respectively. ( b ) Pressure dependence of the volume of CuO. The experimental values, deduced from a Birch–Murnaghan equation of state fitted to data of nanocrystalline CuO up to a pressure of 17 GPa (ref. 21 ), are compared with those calculated by DFT. ( c ) Pressure dependence of the magnetic exchange couplings of CuO. Positive and negative values represent antiferromagnetic and ferromagnetic interactions, respectively. The J’ s in the grey area are ferromagnetic. The uncertainty in the DFT J ij values is between 1.2 and 2.5 meV (that is, smaller than the symbols). Full size image The predictive power of our DFT geometry optimization is confirmed by its capacity to reproduce the volume decrease with pressure as reported up to 17 GPa for nanocrystalline CuO samples [21] . The pressure dependence of the J -values, determined for the optimized atomic structures, compare very well with previous calculations [14] , that use the available experimental structures up to 8.8 GPa (ref. 16 ). Most importantly, J z strongly increases, whereas J 2a is nearly constant for pressures up to ~20 GPa, after which they increase in a similar manner as J z . Of the three smaller J -values, J a is most affected by pressure and becomes ferromagnetic beyond about 2 GPa. The magnetic frustration, that is, the competition between J a and J 2a (ref. 14 ), is therefore strongly enhanced by pressure. The change in ratio between the two largest J -values, that is, J z /J 2a , evidences that the effective magnetic dimensionality is also affected by pressure. As shown in Fig. 2a , the quasi-1D character of the magnetic structure is enhanced for pressures up to 20 GPa but then is reduced. 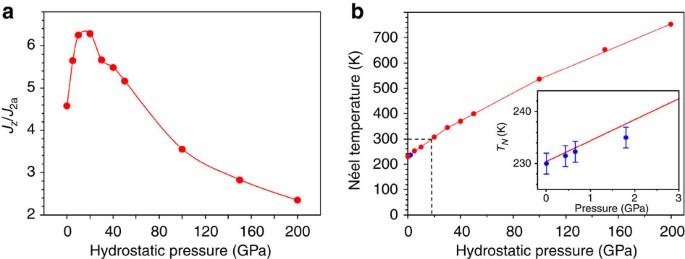Figure 2: High-pressure evolution of the effective magnetic dimensionality and Néel temperature of CuO. (a) Ratio between the two largest magnetic exchange interactions (Jz/J2a). The 1D character of the magnetic structure is first enhanced with pressure (up to 20 GPa) and is then reduced. (b) Pressure dependence of the Néel temperature of CuO. Experimental data (in blue) measured up to 1.8 GPa (ref.23) are compared with the result of the semi-empirical RPA expression (in red) for quasi-1D antiferromagnets22. The inset provides a zoomed view for pressure values smaller than 3 GPa. The experimental error bar23of about ±2 K, estimated from a high-pressure neutron diffraction investigation, is shown using blue bars. Figure 2: High-pressure evolution of the effective magnetic dimensionality and Néel temperature of CuO. ( a ) Ratio between the two largest magnetic exchange interactions ( J z /J 2a ). The 1D character of the magnetic structure is first enhanced with pressure (up to 20 GPa) and is then reduced. ( b ) Pressure dependence of the Néel temperature of CuO. Experimental data (in blue) measured up to 1.8 GPa (ref. 23 ) are compared with the result of the semi-empirical RPA expression (in red) for quasi-1D antiferromagnets [22] . The inset provides a zoomed view for pressure values smaller than 3 GPa. The experimental error bar [23] of about ±2 K, estimated from a high-pressure neutron diffraction investigation, is shown using blue bars. Full size image Pressure effect on the Neel temperature Having determined the pressure dependence of the magnetic exchange coupling constants, we calculate the multiferroic ordering temperature T N up to 200 GPa. We first evaluate it using the semi-empirical random phase approximation (RPA) expression for the quasi-1D AF Heisenberg model on a cubic lattice with intrachain and interchain couplings J and J′ , respectively [22] . The resulting T N is shown in Fig. 2b . Choosing the parameterization such that it reproduces the transition temperature T N =230 K at ambient pressure, we observe a monotonic and substantial increase of T N with pressure. This result coincides with the experimental pressure dependence of T N , as was measured up to 1.8 GPa (ref. 23 ) and reaches RT at ~20 GPa. Pressure effect on the magnetic anisotropy To substantiate this prediction, however, one needs to go beyond the semi-empirical approach. For this purpose, we employed a classical MC technique to explore the competition between the different magnetic states as a function of both pressure and temperature, with the Hamiltonian H=H H +H UA +H DM +H MA , where H H is the Heisenberg exchange, H UA is uniaxial anisotropy (UA), H DM the Dzyaloshinskii Moriya (DM) term and H MA is the multiaxial (MA) anisotropy term. All these terms are relevant, but in particular the anisotropy terms are shown by our DFT calculations to be crucial for describing the effects of pressure. The relevant magneto-crystalline anisotropy energies (MAEs) of CuO have been calculated for the ground-state (GS) AF 1 magnetic structure with MAE=E[uvw]–E[010], where E[uvw] is the energy deduced from spin–orbit (SO) calculations with the magnetization along the [uvw] crystallographic direction. 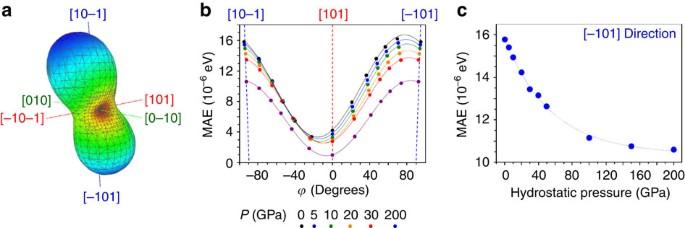Figure 3: High-pressure evolution of the magneto-crystalline anisotropy of CuO. MAE of CuO calculated for the GS AF1magnetic structure7where MAE=E[uvw]–E[010] andE[uvw] is the energy deduced from SO calculations with magnetization along the [uvw] crystallographic direction. (a) The three-dimensional shape of MAE shows that the easy axis of magnetization at 0 GPa is thebaxis, that is, [010] direction of the crystallographic cell. (b) MAE in the plane normal to thebaxis, which is reduced by pressure. (c) Exponential decay of MAE with pressure, as illustrated for the [−101] direction. Figure 3a shows the anisotropy energy surface [24] for CuO in the AF 1 magnetic order at a pressure of 0 GPa. Two minima are observed along the [010] direction and equivalently [0–10] direction. Thus, the SO DFT calculations properly predict that the b axis is the easy axis of magnetization of CuO for the low-T magnetic phase AF 1 . A similar result is obtained for the entire pressure domain, that is, from 0 to 200 GPa. However, the MAE values are rapidly decreasing with pressure as evidenced in Fig. 3b , in which the MAE in the (a,c) plane is plotted as a function of the angle ϕ , such that ϕ=0 ° corresponds to the [101] direction. It also turns out that the hardest axis of magnetization (largest MAE value) is close to the [10–1] direction, that is, the antiferromagnetic direction. The pressure dependence of the MAE approximately follows an exponential decay, as is illustrated in Fig. 3c for the [−101] direction. Figure 3: High-pressure evolution of the magneto-crystalline anisotropy of CuO. MAE of CuO calculated for the GS AF 1 magnetic structure [7] where MAE= E [uvw]– E [010] and E [uvw] is the energy deduced from SO calculations with magnetization along the [uvw] crystallographic direction. ( a ) The three-dimensional shape of MAE shows that the easy axis of magnetization at 0 GPa is the b axis, that is, [010] direction of the crystallographic cell. ( b ) MAE in the plane normal to the b axis, which is reduced by pressure. ( c ) Exponential decay of MAE with pressure, as illustrated for the [−101] direction. Full size image Pressure effect on the electronic polarization Before discussing the MC data, we can estimate the order of magnitude of the ferroelectric polarization, P , by using the empirical formula proposed by Katsura et al. [25] : P =( V/Δ ) 3 , where V is the Cu–O electronic overlap integral and Δ is the p–d splitting. The superexchange parameter is approximately given by, J = V 4 / Δ 3 . The relevant superexchange interactions for the ferroelectric nature of CuO are J a and J b . Therefore, taking J =5 meV and Δ =1.4 eV (refs 7 , 26 ), we find P =0.15 μC cm −2 , which is close to the experimental value [27] of about 0.1 μC cm −2 . Alternatively, we can estimate the ferroelectric polarization directly from our DFT calculations using the Berry phase method [28] . As previously demonstrated theoretically [8] , the lattice contribution to the polarization ( P l ) is small compared with the electronic one ( P e ) in CuO, that is, P l ~0.050 μC cm −2 and P e ~0.200 μC cm −2 . Here, taking into account the SO coupling, P e was calculated to be 0.286 μC m −2 at 0 GPa. It should be noted that we find an electronic polarization along the b direction ( P e ~0 along a and c directions), in good agreement with the experiments. To determine the pressure effect on the value of P e , we have considered two other pressure values, that is, 20 and 40 GPa. Our calculations show that P e =0.286, 0.379 and 0.455 μC cm −2 at 0, 20 and 40 GPa, respectively, and at zero temperature. These polarization values are along the b direction, and under pressure the polarization along the a and c directions remains zero. This clearly confirms that applying pressure on CuO leads to an increase of the electric polarization, which is predicted to be along the b direction only. The finite temperature MC simulations use the J -values obtained from the DFT calculations and, in particular, incorporate the H MA term that is rapidly decreasing with pressure. 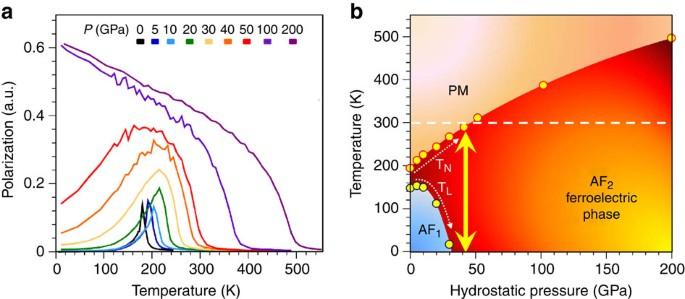Figure 4: Temperature–pressure phase diagram of the magnetic model of CuO. Magnetic and ferroelectric properties of CuO as determined by MC calculations, based on the microscopic magnetic interactions. (a) Temperature dependence of the ferroelectric polarization, which is proportional to the calculated spin current, for different values of hydrostatic pressure. (b) Temperature–pressure magnetic phase diagram of CuO. The RT is indicated by the horizontal white dashed line and the giant stabilization of the AF2ferroelectric phase of CuO is highlighted by the vertical yellow double arrow. PM stands for paramagnetic. Figure 4a shows the resulting spin current as a function of pressure, which is a quantity that is directly proportional to P . We observe that at ambient pressure close to the paramagnetic to AF1 transition, a spontaneous polarization is induced. This polarization is found to be non-zero between T N =200 and T L =150 K, which compares well with the experimentally observed stability domain of the incommensurate AF 2 magnetic order, between T N =230 and T L =213 K. Figure 4: Temperature–pressure phase diagram of the magnetic model of CuO. Magnetic and ferroelectric properties of CuO as determined by MC calculations, based on the microscopic magnetic interactions. ( a ) Temperature dependence of the ferroelectric polarization, which is proportional to the calculated spin current, for different values of hydrostatic pressure. ( b ) Temperature–pressure magnetic phase diagram of CuO. The RT is indicated by the horizontal white dashed line and the giant stabilization of the AF 2 ferroelectric phase of CuO is highlighted by the vertical yellow double arrow. PM stands for paramagnetic. Full size image The fact that the calculated values are somewhat lower than the experimental ones is due to the model approximations involved and indicates that the MC results are conservative in the sense that they rather tend to underestimate the stability of the multiferroic phase. When the pressure is increased the polarization grows, in agreement with our DFT result for P e dependence with pressure, and extends to a larger temperature range. For instance, at 30 GPa an increase of about 20% is observed with respect to the polarization at 0 GPa, and the temperature range is larger and in between 245 and 115 K. At 200 GPa, the multiferroic phase (AF 2 ) extends down to zero temperature and the ferroelectric polarization is more than doubled. The MC results confirm the increase of T N with pressure, in accordance with the experimental observations for pressures up to 2 GPa and the results from the semi-empirical RPA expressions. We find good quantitative agreement for the values of the differential pressure increase of T N from experiment, 2.7 (0.2) K GPa −1 (ref. 23 ), and from the RPA and MC results, 3.5 (0.3) K GPa −1 and 3.0 (0.3) K GPa −1 , respectively. The calculated temperature–pressure phase diagram of CuO (see Fig. 4b ) shows, in addition, a monotonic decrease of T L with pressure. As a consequence, the non-polar AF 1 phase disappears from the phase diagram with increasing pressure, at the benefit of the multiferroic AF 2 phase. The MC simulations indicate that T N reaches RT at ~40 GPa, which is higher than the ~20 GPa, obtained from the semi-empirical RPA expressions, underlining that the MC pressure of ~40 GPa is a conservative estimate for the critical pressure value. Finally, the present temperature–pressure phase diagram of CuO evidences under high pressure a large increase of the stability range of the incommensurate multiferroic AF 2 phase, which is stable in a domain of only 20 K (from 210 to 230 K) at 0 GPa, and in a domain larger than 300 K (from 0 to T> 300 K) at 20–40 GPa. Such a giant stabilization of a multiferroic phase by pressure has never been observed or proposed. Indeed, except for CuO, all the reported pressure–temperature phase diagrams of multiferroic materials (Ni 3 V 2 O 8 , MnWO 4 , TbMnO 3 and RMn 2 O 5 with R=Tb, Dy, Ho…) [29] , [30] , [31] , [32] lead to the same conclusion, namely that the stability range of the incommensurate magnetic phase is reduced by pressure. The fact that our theoretical and predictive approach correctly reproduces the experimental low-pressure results gives considerable credit to our predictions. In contrast to the multiferroic compounds mentioned above, the geometrical modifications (bond distances and angles) under pressure in CuO induce an increase of the magnetic frustration, as previously demonstrated up to 8.8 GPa (ref. 14 ) and confirmed here for a larger pressure domain from 0 to 200 GPa. Further theoretical efforts on the dependence of the magnetic frustration versus pressure (chemical or physical) in CuO and the related compounds is clearly needed and will be of direct interest in the quest of type-II multiferroics with tunable ferroelectric and magnetic properties. The first RT binary multiferroic material is thus within reach: CuO at pressures of 20–40 GPa. To be practical, for technical applications, the high-pressure form of CuO must be made stable at ambient conditions. To achieve this, there are at least two strategies. Very special for CuO is the possibility to stabilize its high pressure form at a nanoscale level by applying high-energy ion irradiation at high pressures [33] . In such experiments, the quenched high-pressure structure remains even after releasing pressure. Another promising strategy can be a core-shell synthesis [34] according to which CuO nanoparticles are embedded in a shell material that has a negative thermal expansion coefficient, which then acts as an effective pressure medium for the CuO core. DFT calculations The DFT calculations have been carried out by using two different codes: Vienna Ab initio Simulation Package (VASP) [35] for the geometry optimization at the different pressure values and WIEN2k programme package [36] for the calculation of the magnetic exchange, J ij , and magneto-crystalline anisotropy energy, MAE, values. For the geometry optimizations, a 16 formula units cell has been used, that is, 2a × 2b × 2c, with a, b and c being the crystallographic cell parameters. The GS magnetic order (AF 1 ) has been considered for the geometry optimization. The parameters used in the VASP calculations are the following. We have used the GGA+U approach with U eff =6.5 eV for the Cu(3d) states, as in our previous investigation [8] , [20] . It allows having a proper description of the structural properties of CuO. The wave functions are expanded in a plane wave basis set with kinetic energy below 500 eV. The VASP package is used with the projector augmented wave method of Blöchl [37] . The integration in the Brillouin Zone is done by the Methfessel–Paxton method [38] on a 3 × 3 × 3 set of k -points determined by the Monkhorst–Pack scheme [39] . All atoms were then allowed to relax by following a conjugate gradient minimization of the total energy scheme (3 × 10 −2 eV Å −1 ). The magnetic exchange parameters ( J ij values) were estimated based on the optimized atomic structures and for each pressure (from 0 to 200 GPa), and using the WIEN2k programme package with the onsite PBE0 (ref. 40 ) hybrid functional for 8 and 32 f.u. cells. The J ij values have been deduced from a least-squares fit procedure and the quality of the fits is shown in Fig. 5a,b . It should be noticed that the choice of the PBE0 onsite hybrid functional in WIEN2k was motivated by its ability to properly reproduce the magnetic exchange coupling in a series of copper oxide compounds and its dependence with the Cu–O–Cu bond angle [14] . 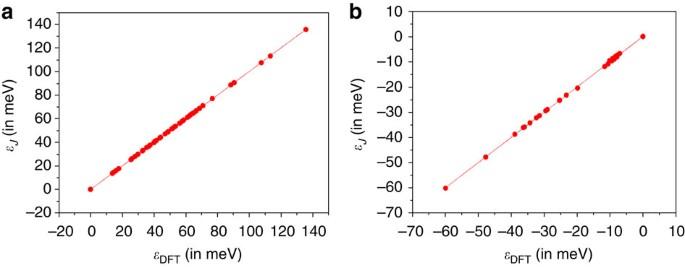Figure 5: Quality of the DFT magnetic exchange parameters. Graphical representation of the quality of the least-squares fit procedure for the 8 (a) and 32 (b) formulae units models.εDFTandεJare, respectively, the relative energies (with respect to AF1) deduced from the DFT calculations and theJparameters. The s.d. values are 0.12 and 0.25 meV, respectively, for the 8 and 32f.u.models. Figure 5: Quality of the DFT magnetic exchange parameters. Graphical representation of the quality of the least-squares fit procedure for the 8 ( a ) and 32 ( b ) formulae units models. ε DFT and ε J are, respectively, the relative energies (with respect to AF 1 ) deduced from the DFT calculations and the J parameters. The s.d. values are 0.12 and 0.25 meV, respectively, for the 8 and 32 f.u. models. Full size image The MAE value has been estimated for the AF 1 GS magnetic structure, using the code WIEN2k with the PBE0 hybrid functional and including the SO coupling. MAE corresponds to an energy difference between two directions of the magnetization density. Here we use the [010] direction, that is, the easy axis, as the reference: E[uvw] is the energy deduced from SO calculations with magnetization along the [uvw] crystallographic direction. It should be noticed that MAE is very sensitive to the k -mesh. The quality of the k -mesh has been carefully chosen, leading to the use of a 5 × 12 × 6 set of k -points for the 8 f.u. cell. The electronic contribution ( P e ) to the polarization P was evaluated using the Berry phase approach [28] . As previously shown [8] , the lattice contribution ( P l ) is small compared with the electronic one ( P e ) in CuO: P e ~0.200 μC cm −2 and P l ~0.050 μC cm −2 . Here we have redone such calculations using the VASP code with the GGA+U formalism and a U eff value of 7.5 eV, to match the J ij values obtained using the PBE0 hybrid functional in our WIEN2k calculations. The non-collinear magnetic structure, AF 2 , previously discussed in ref. 8 has been used. To have adequate electric polarization values, it was crucial to turn on the SO coupling during the structural relaxation. Indeed, at 0 GPa, P e =0.053 and 0.286 μC cm −2 , respectively, for the atomic structure relaxed without and with SO. Estimation of T N based on the RPA formula The above equation has been developed for the estimation of T N of a quasi-1D AF Heisenberg model on a cubic lattice with J and J′ , the intrachain and interchain couplings, respectively [22] . The related GS magnetic order leads to the following energy expression: Although CuO is a quasi-1D magnetic system, it exhibits a more complex magnetic order due to the low symmetry of its atomic structure (monoclinic space group: C2/c). As a consequence, its GS magnetic order (AF 1 ) leads to the following energy expression: with J 2a being the predominant super-superexchange interaction. For more details, see (refs 7 and 20 ). Considering E (GS)= E (AF 1 ) and J z as the intrachain coupling, that is, J z =J , we can define J′ as: Our detailed results are illustrated in Fig. 6 . 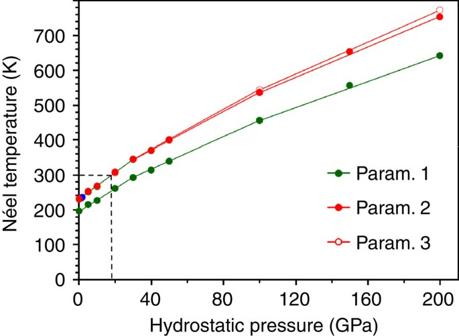Figure 6: High-pressure evolution of the Néel temperature of CuO. Pressure dependence of the Néel temperature of CuO. Experimental data measured up to 1.8 GPa are compared with theoretical ones deduced from an analytical expression developed for S=1/2 quasi-1D Heisenberg antiferromagnets22. Three parameterizations are used, the original one withc=0.233 andα=2.6 (param.1) and two modified forms, withc=0.284 andα=2.6 (param.2) and withc=0.233 andα=8.4 (param.3). The black dash line evidences thatTNis reaching RT at about 20 GPa (from both param. 2 and 3). Figure 6: High-pressure evolution of the Néel temperature of CuO. Pressure dependence of the Néel temperature of CuO. Experimental data measured up to 1.8 GPa are compared with theoretical ones deduced from an analytical expression developed for S=1/2 quasi-1D Heisenberg antiferromagnets [22] . Three parameterizations are used, the original one with c =0.233 and α =2.6 (param.1) and two modified forms, with c =0.284 and α =2.6 (param.2) and with c =0.233 and α =8.4 (param.3). The black dash line evidences that T N is reaching RT at about 20 GPa (from both param. 2 and 3). Full size image Classical MC simulations The model Hamiltonian used in MC simulations is given by, where, H H is the Heisenberg part, H UA is UA term, H DM is DM term and H MA is the MA anisotropy. The Heisenberg term and the UA term can be written together as, where refer to exchange parameters at pressure P . The various exchange parameters are J z , J x , J 2a , J a and J b (see Fig. 1a ). The UA term has been included in the Heisenberg part by making the following replacement: This allows a lower energy for a collinear AF 1 state in which all the spins are aligned along the y axis. The DM term is given by As we are mainly interested in the competition between two magnetic states, the collinear AF 1 and the non-collinear AF 2 , we restrict the spins to reside in y–z plane only. Therefore, we only introduce a DM vector pointing along x direction. The experimental observation that the AF 2 state is stable in a narrow temperature window between 230 and 213 K is reproduced in an effective manner by introducing a MA anisotropy term, in the Hamiltonian of the form [24] , The Heisenberg term, H H , alone leads to a degeneracy of GSs. The GS manifold consists of perfectly ordered, interpenetrating sub-lattices with vector order parameters whose relative orientation is left completely undetermined by the Heisenberg term alone. The UA term prefers a collinear magnetic state, where the two sub-lattice order parameters align along the y axis. This is precisely the experimentally observed AF 1 state of CuO. The DM coupling favours a non-collinear (but coplanar) state and, therefore, it competes with the H UA . There is a critical strength of the DM coupling, D c , above which the AF 1 is not the GS. Given that the AF 1 is the GS at ambient pressure, we conclude that D<D c . We use the Metropolis algorithm to perform Markov Chain MC simulations on classical spins. The simulations are started with a completely random spin configuration at high temperature. Because of the presence of many competing interactions and nearly degenerate GSs, the simulations require a large number of equilibration and averaging steps. We use ~10 6 MC steps for equilibration and a similar number of steps for averaging at each temperature. The temperature is then reduced in small steps (~5 K) and the system is allowed to anneal towards the GS spin configuration. The main quantity of interest is the spin current, which is defined as ‹ e ij × ( S i × S j )›,where e ij is a vector connecting spins S i and S j , and the angular brackets denote thermal as well as spatial average. The ferroelectric polarization is proportional to the spin current with a prefactor estimated to be 0.150 μC cm −2 following Katsura et al. [25] The simulations are carried out on lattices with N =12 3 sites. We have checked the stability of our results for larger sizes (up to N =32 3 ) for selected values of pressure ( Supplementary Fig. S1 ). The procedure used to estimate T L and T N for 2 pressures (0 and 30 GPa) is shown in Fig. 7 . 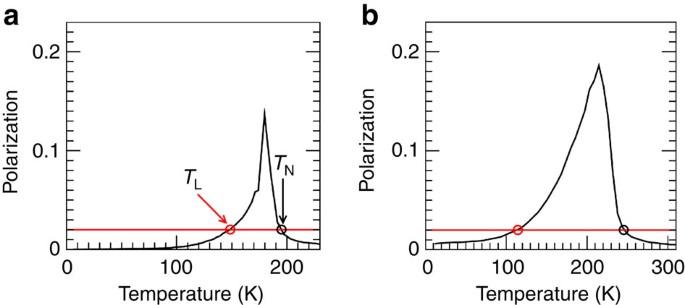Figure 7: Temperature dependence of the spin current. The spin current is proportional to ferroelectric polarization and is given for two sets of parameters corresponding toP=0 GPa (a) andP=30 GPa (b). An increase in spin current upon decreasing temperature is an indication of the onset of a non-collinear ferroelectric phase. The decrease of spin current below a cutoff value is defined at the transition to a collinear state. We show the red horizontal line (P=0.02) as the cutoff value used for inferringTNandTL. Figure 7: Temperature dependence of the spin current. The spin current is proportional to ferroelectric polarization and is given for two sets of parameters corresponding to P =0 GPa ( a ) and P =30 GPa ( b ). An increase in spin current upon decreasing temperature is an indication of the onset of a non-collinear ferroelectric phase. The decrease of spin current below a cutoff value is defined at the transition to a collinear state. We show the red horizontal line ( P =0.02) as the cutoff value used for inferring T N and T L . Full size image The UA parameter λ =0.02 is kept constant. The MA anisotropy B decreases exponentially with increasing pressure; we use B =500 e − P /10 ( B =500 for P =0 and B =24.9 for P =30). The exponential decrease is motivated by the DFT results presented in Fig. 3 . The large value of B at P =0 is required to obtain the narrow range of stability of AF 2 state at high temperatures. Although UA term is also decreasing with pressure, this does not lead to any crucial changes in the phase diagram shown in Fig. 4 . We also keep the DM coupling fixed to D =0.8 D c . The choice of the parameter D is not very crucial, as long as D is smaller than D c . To illustrate this point, we show the results for spin current for various values of D at P =0 GPa and P =30 GPa in Supplementary Fig. S2 . How to cite this article: Rocquefelte, X. et al. Room-temperature spin-spiral multiferroicity in high-pressure cupric oxide. Nat. Commun. 4:2511 doi: 10.1038/ncomms3511 (2013).